Human hypocretin and melanin-concentrating hormone levels are linked to emotion and social interaction The neurochemical changes underlying human emotions and social behaviour are largely unknown. Here we report on the changes in the levels of two hypothalamic neuropeptides, hypocretin-1 and melanin-concentrating hormone, measured in the human amygdala. We show that hypocretin-1 levels are maximal during positive emotion, social interaction and anger, behaviours that induce cataplexy in human narcoleptics. In contrast, melanin-concentrating hormone levels are minimal during social interaction, but are increased after eating. Both peptides are at minimal levels during periods of postoperative pain despite high levels of arousal. Melanin-concentrating hormone levels increase at sleep onset, consistent with a role in sleep induction, whereas hypocretin-1 levels increase at wake onset, consistent with a role in wake induction. Levels of these two peptides in humans are not simply linked to arousal, but rather to specific emotions and state transitions. Other arousal systems may be similarly emotionally specialized. Because of the link between the loss of hypocretin (Hcrt) neurons and human narcolepsy [1] , [2] , [3] , much work has focused on Hcrt’s putative role in maintaining waking. Its role in preventing cataplexy has remained unclear. Moreover, studies using Fos immunohistochemistry, Hcrt knockouts and Hcrt receptor blockers have suggested conflicting conclusions about the relation of Hcrt to food intake, anxiety, stress, positive versus negative emotions and muscle tone increase versus muscle tone decrease [4] , [5] . Some of these conflicts may stem from the limited temporal resolution of the Fos technique, which reflects activity occurring over the entire 2-h period before killing. Others may be due to species differences and the brain reorganization that occurs in Hcrt mutant animals [6] . Cataplexy, a sudden loss-of-muscle tone with maintained consciousness, is the unique symptom of narcolepsy. Triggers for cataplexy are strikingly species-specific. In human narcoleptics, cataplexy is most commonly triggered by laughter, next most commonly by angry interactions, less frequently by athletic exertion and rarely by eating, pain or anxiety [7] . In the narcoleptic sheep, cataplexy is most reliably triggered by the sound of dogs barking or by being knocked over, presumably anxiety-eliciting stimuli, but never by eating or by playing behaviour (our unpublished observations and [8] ). In narcoleptic dogs, cataplexy is triggered by eating favoured foods or by ‘playful’ running and pulling, never by aversive situations [6] . In narcoleptic cattle, aggressive behaviour in the affected animal is the most frequent trigger [9] . In ‘narcoleptic’ rats and mice, exploration and the eating of certain foods are the most reliable triggers of cataplexy [10] . Although the activity of Hcrt cells may have a role in preventing cataplexy, these neurons are not solely active during behaviours associated with cataplexy, a symptom which typically happens less than once or twice a week in most human narcoleptics. In the normal rat, Hcrt neurons discharge at variable rates throughout the waking period [11] and release of this peptide, measured in cats, varies considerably across the waking state [12] . Hcrt unit discharge rate, observed in rats is minimal in non-rapid eye movement sleep. Although rates are low in rapid eye movement sleep, occasional burst discharge of Hcrt cells is seen during this state [11] , [13] . The functional role of melanin-concentrating hormone (MCH) is also unclear. MCH is synthesized in non-Hcrt neurons that are anatomically intermixed with Hcrt neurons, and these neurons are thought to interact [2] , [14] , [15] , [16] . Although most evidence suggests that Hcrt neurons are maximally active during waking, similar evidence suggests that MCH neurons are maximally active during sleep [17] , [18] . The release of MCH across the sleep–wake cycle and its relation to waking behaviour has not been measured in any species. In the current paper, we first report on the levels of Hcrt-1 and MCH in the rat, showing that these levels are synchronously modulated in the amygdala and hypothalamus, increasing the likelihood that measurements of levels of these peptides in the human amygdala reflect release in widespread brain regions. We then report measurements of Hcrt-1 and MCH levels in the amygdala of human patients, each monitored continuously over several days during their complete range of spontaneous behaviours and with their assistance in quantifying their emotions. We find that maximal Hcrt levels occur during social interactions and subject-reported positive emotions or anger. Minimal Hcrt levels occur during pain and sleep. MCH levels are maximal at sleep onset and after eating. Minimal MCH levels occur during waking pain and during social interaction. This is the first study of neurotransmitter levels in relation to human emotions. Hcrt-1 and MCH levels in the rat brain Hcrt neurons produce both Hcrt-1, which is stable, and Hcrt-2, which is rapidly metabolized. Both peptides are derived from preprohypocretin [19] , [20] . We first undertook studies of Hcrt-1 and MCH levels in four rats to determine whether there were strong regional differences between levels in the hypothalamus, the location of all Hcrt and most MCH cell bodies, and the amygdala, one of the many brain regions innervated by collaterals of Hcrt and MCH axons, and the region sampled in all of our human subjects, as dictated by clinical considerations. In the rat, average waking Hcrt-1 concentrations were 0.11±0.02 fmol per 10 μl in the hypothalamus and 0.06±0.01 fmol per 10 μl in the amygdala. Average waking MCH concentrations were 0.10±0.03 fmol per 10 μl in the hypothalamus and 0.10±0.03 fmol per 10 μl in the amygdala. Hcrt-1 levels in the hypothalamus were highly correlated with Hcrt-1 levels in the amygdala. 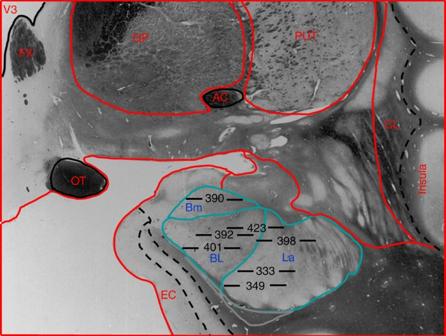Figure 1: Location of microdialysis probes in human subjects. Placements of membranes at the tip of each probe are labelled by subject number. Horizontal lines on either side of each subject number are to scale, and their total length indicates the 5-mm area sampled by each membrane. The position of each membrane in the amygdala is drawn to scale. The anatomic outline graphic was adapted from the human brain atlas by Maiet al.58. AC, anterior commissure; BL, basolateral nucleus of the amygdala; Bm, basomedial nucleus of the amygdala; CL, claustrum; EC, entorhinal cortex; FX, fornix; GP, globus pallidus; La, lateral nucleus of the amygdala; OT, optic tract; PUT, putamen; V3, third ventricle. MCH levels in the hypothalamus were also highly correlated with MCH levels in the amygdala ( Table 1 ). Table 1 Rat number and correlation of Hcrt and MCH levels in the hypothalamus and amygdala. Full size table Microdialysis setup in human patients All eight patients were psychologically normal and had seizures of suspected unilateral temporal lobe origin. Patients were implanted with bilateral probes to localize the side which contained the primary seizure focus for subsequent surgical removal. Using angiography and magnetic resonance imaging, electrode trajectory was adjusted to avoid major blood vessels. Electrodes generally passed though the temporalis muscle, and dialysis probes were all in the amygdala ( Fig. 1 ). Some patients reported episodic pain localized to the muscle, whereas others did not have significant pain. Microdialysis experiments were performed between 2 and 5 days after electrode implantation. Only one patient had a seizure during the period in which we collected the dialysate. No data from the 5-h period after seizure onset was used in the current study. 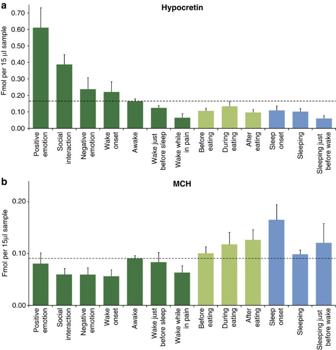Figure 2: Hcrt and MCH levels across waking and sleep activities. (a) Maximal Hcrt levels in waking are seen during positive emotions, social interactions and awakening, minimal levels are seen before sleep and while reporting pain. Changes during and after eating are smaller than those during monitored non-eating-related activities. Waking values in shades of green, sleep values in shades of blue. Awake indicates samples in which subjects were awake, but were not exhibiting social interaction or reporting emotion. (b) Maximal MCH levels are seen at sleep onset and after eating. Minimal levels are seen during wake onset, social interaction and pain. Error bars represent ±s.e.m. Primary seizure foci were found to be in ipsilateral or contralateral cortical regions (see Table 2 ). Figure 1: Location of microdialysis probes in human subjects. Placements of membranes at the tip of each probe are labelled by subject number. Horizontal lines on either side of each subject number are to scale, and their total length indicates the 5-mm area sampled by each membrane. The position of each membrane in the amygdala is drawn to scale. The anatomic outline graphic was adapted from the human brain atlas by Mai et al . [58] . AC, anterior commissure; BL, basolateral nucleus of the amygdala; Bm, basomedial nucleus of the amygdala; CL, claustrum; EC, entorhinal cortex; FX, fornix; GP, globus pallidus; La, lateral nucleus of the amygdala; OT, optic tract; PUT, putamen; V3, third ventricle. Full size image Table 2 Patient information and parameters of implanted electrodes. Full size table Continuously recorded videos were scored for TV watching, social interactions (talking to physicians, nursing staff or family), eating, pain reports, clinical manipulations and sleep–wake transitions. Notes of activities were made throughout the study, every 15 min in synchrony with our 15-min microdialysis-sample collection interval, by an experimenter in the patients’ room. The subjects rated their moods and attitudes on our questionnaire, administered every hour during waking (see Supplementary Methods ). Hcrt-1 and MCH levels in the human brain Average waking (Awake, Fig. 2 ) Hcrt-1 concentration in samples from the amygdala of humans was 0.16±0.01 fmol per 15 μl. Average waking MCH concentration was 0.09±0.01 fmol per 15 μl. We compared levels in our 15-min microdialysis samples from the left and right amygdala of two patients to determine whether changes in the levels of these peptides were bilaterally correlated. Hcrt-1 levels in the right and left amygdala were significantly correlated in the 24-h period monitored in both patients, as were MCH levels (Patient 4; Hcrt-1, r =0.81, P =0.0001, df=77; MCH, r =0.40, P =0.0003, df=77; Patient 5: Hcrt-1, r =0.60, P =0.0001, df=76; MCH, r =0.22, P =0.048, df=76, Pearson’s product–moment correlation coefficient). All the data presented below were derived from the left amygdala. Figure 2: Hcrt and MCH levels across waking and sleep activities. ( a ) Maximal Hcrt levels in waking are seen during positive emotions, social interactions and awakening, minimal levels are seen before sleep and while reporting pain. Changes during and after eating are smaller than those during monitored non-eating-related activities. Waking values in shades of green, sleep values in shades of blue. Awake indicates samples in which subjects were awake, but were not exhibiting social interaction or reporting emotion. ( b ) Maximal MCH levels are seen at sleep onset and after eating. Minimal levels are seen during wake onset, social interaction and pain. Error bars represent ±s.e.m. Full size image Hcrt-1 and MCH levels correlate with emotional state After log transformation, one-way analysis of variance of peptide levels measured during the 13 behaviours evaluated showed significant differences for both Hcrt-1 ( F =7.4, P <0.0001) and MCH ( F =3.4, P <0.001). 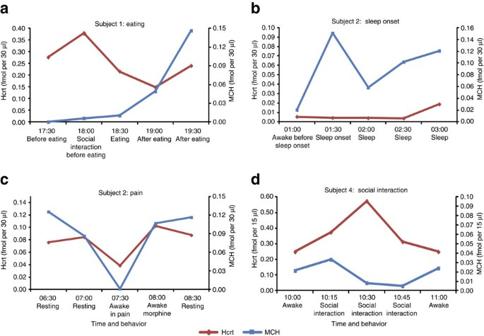Figure 3: Examples of single-case raw data on Hcrt and MCH release from individual patients. Release pattern over time shows that (a) MCH levels increase after eating, (b) MCH levels increase at sleep onset, (c) both Hcrt and MCH levels are low during pain and (d) Hcrt levels increase with social interaction. With the exception of the example shown inc, all data in this study were collected during morphine-free periods. SeeFig. 2for average levels in each condition. The number of observations for the analysis of variances and Fisher’s least significant difference post-hoc comparisons are provided in Table 3 . We found that high levels of Hcrt-1 in humans consistently occurred during social interactions ( P <0.002), comparing the mean Hcrt-1 levels during social interaction with awake levels (awake=waking without social interaction or emotion reports; Figs 2a , 3d and 4 ). Waking periods with positive emotion had significantly higher levels of Hcrt-1 than waking periods with negative emotion ( P <0.02; Fig. 2a ). Table 3 Measurements of Hcrt and MCH levels across behaviours. Full size table Figure 3: Examples of single-case raw data on Hcrt and MCH release from individual patients. Release pattern over time shows that ( a ) MCH levels increase after eating, ( b ) MCH levels increase at sleep onset, ( c ) both Hcrt and MCH levels are low during pain and ( d ) Hcrt levels increase with social interaction. With the exception of the example shown in c , all data in this study were collected during morphine-free periods. See Fig. 2 for average levels in each condition. 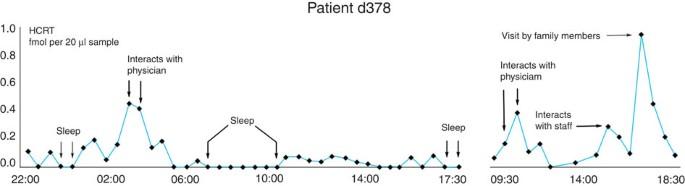Figure 4: Time course of Hcrt release over a 20-h period in patient d378. A Hospal dialysis membrane was used in this subject who was therefore not used in the statistical comparisons with the other seven subjects. However, the results with these two membrane types were indistinguishable. Hcrt release is minimal during sleep and maximal during periods of social interaction. Full size image Figure 4: Time course of Hcrt release over a 20-h period in patient d378. A Hospal dialysis membrane was used in this subject who was therefore not used in the statistical comparisons with the other seven subjects. However, the results with these two membrane types were indistinguishable. Hcrt release is minimal during sleep and maximal during periods of social interaction. Full size image Average Hcrt-1 levels in the 15-min period of wake onset ( Fig. 2a ) were significantly higher than levels during sleep ( P <0.01) and during the 15-min wake period before sleep ( P <0.05). Surprisingly, average Hcrt-1 values during periods of waking pain were as low as sleep values ( Figs 2a and 3c , and Table 3 ). MCH levels were significantly increased after eating compared with awake levels ( P <0.01; Figs 2b and 3a ). We found an interesting dissociation between Hcrt-1 and MCH levels at sleep onset. Hcrt-1 levels did not significantly change at sleep onset, because Hcrt-1 levels were reduced before sleep onset and remained below awake levels throughout sleep ( P <0.01, Fig. 2a ). Conversely, the MCH level was maximal at sleep onset ( Figs 2b and 3b ) and this value significantly exceeded wake onset levels ( P <0.01). We found a significant negative relation between MCH levels and the level of questionnaire-indicated pain ( r =−0.32, df=45, P =0.03). There was also a significant positive correlation between Hcrt-1 levels and the level of questionnaire-indicated anger ( r =0.49, df=45, P =0.043), consistent with anger being a common trigger of human cataplexy [7] . In the current study we found that Hcrt-1 level is not a simple function of arousal. Hcrt-1 levels were higher when subjects showed laughter or excitement than when subjects reported feeling frustrated or sad. Furthermore, we found that Hcrt levels were low during waking pain. Allowing for species differences, these human data bear considerable resemblance to data on Hcrt cell activity in animals. Our prior studies of Fos expression, an indication of elevated rates of neuronal discharge, in the Hcrt neurons of wild-type mice found that these neurons are maximally active during performance of rewarded behaviours [5] , and that Hcrt knock-out mice were strikingly deficient in staying awake to perform rewarded behaviours. Two other studies reported a similar involvement of Hcrt neurons in positive reinforcement [21] , [22] . Our studies of Fos expression in wild-type mice also showed that Hcrt neurons were not activated beyond baseline levels during foot shock, or foot-shock avoidance behaviour, despite high levels of electroencephalography (EEG) arousal [5] . We have also reported that Hcrt unit activity in rats is suppressed in novel situations eliciting withdrawal, despite maximal levels of EEG activation. In contrast, Hcrt unit activity is high during grooming and exploration [11] . In studies in normal dogs, we found that treadmill running does not elevate Hcrt level, whereas play behaviour of similar cardiovascular intensity greatly increases the Hcrt level [23] , [24] . Our prior studies of Fos expression in animals in combination with our current results in humans suggest the Hcrt system promotes arousal associated with positive emotion and anger, rather than arousal in general. The amygdala is known to be a vital structure in sleep regulation [25] , [26] , [27] , [28] , [29] , [30] . We have found sleep-active and cataplexy-active neurons in the amygdala of narcoleptic dogs [25] and evidence that pathology in the amygdala is linked to the symptoms of canine narcolepsy [29] . However, the pattern of Hcrt-1 release that we see in the amygdala is unlikely to be restricted to the amygdala. The branching pattern of individual Hcrt neurons [31] suggests that a similar pattern of release is likely to be observed in all target regions. In prior investigations of arousal-related systems with similar widely branching axons, we and others have found, for example, that serotonin, norepinephrine and dopamine release in the spinal cord are highly correlated with release in the brainstem [32] . In a prior study we have found that Hcrt release follows the same profile in the hypothalamus and the brainstem locus coeruleus [12] , and in the current study we see the same pattern in the amygdala and hypothalamus of rats. Humans who have attempted suicide have reduced levels of Hcrt-1 in their cerebrospinal fluid (CSF) [33] . Furthermore, a study of the performance of depressed humans in a structured task found that although they work as hard as non-depressed individuals to avoid loss of money, they do not work as hard as controls to acquire additional money [34] . This parallels our animal studies showing activation of Hcrt neurons during positively motivated tasks, but not during negatively motivated tasks [5] . The current results, in concert with these prior animal and human studies, suggest that depression and reported difficulties with social interaction in narcolepsy and Parkinson’s [35] may be related to the loss of Hcrt cells in both of these conditions [2] , [14] , [36] . However, we cannot eliminate the indirect role of the disability that accompanies these disorders in generating depression in humans. Our data suggest that Hcrt antagonism may be a risk factor for depression and that Hcrt supplementation may have antidepressant effects. We found that Hcrt levels do not decrease significantly at sleep onset. This suggests that a reduction in Hcrt-1 level may be linked to the quiet waking that precedes sleep, rather than being directly linked to sleep onset. Furthermore, our findings of low levels of Hcrt during pain in humans and low levels of Hcrt unit activity during anxiety in rats and mice [5] , [11] suggest that Hcrt antagonists, now being developed as hypnotic agents [37] , may not be effective in sleep induction in insomnia resulting from these aversive conditions, as the current data suggest that activity of the Hcrt system is already minimal at these times. On the other hand, our finding that MCH levels are maximal at sleep onset suggests that stimulation of the MCH system may alleviate insomnia. Although we did not find that Hcrt-1 levels significantly decreased at sleep onset, Hcrt-1 levels showed a substantial increase at awakening. This is consistent with our prior work in rats showing that Hcrt neurons burst before awakening [11] and with the finding that optogenetic activation of Hcrt cells can induce waking in mice [38] . Increased activity at wake onset, however, is not confined to the Hcrt neurons, but is also seen in medial reticular [39] noradrenergic, serotonergic [40] , histaminergic and other neurons [39] . The concept of an ascending activating system and the subsequent realization that there are several components to this system led to suggestions that these systems worked in concert and redundantly, that is, the cholinergic, adrenergic, histaminergic and hypocretinergic systems were active simultaneously to sustain waking [41] . The current results suggest the existence of a substantial level of specialization for the Hcrt system and perhaps for other traditionally designated ‘arousal systems’. The minimal level of Hcrt-1 during pain indicates that other, as yet unidentified, systems must be responsible for pain-induced arousal in humans. Narcoleptics have been reported to be hyperalgesic [42] . A large amount of data has suggested, but not proved, a reciprocal relationship between the activity of MCH cells and Hcrt cells [15] , [43] , [44] , [45] . Our data are not inconsistent with the general idea of a reciprocal relationship. We see high levels of Hcrt-1 in relation to social activity and emotion, particularly positive emotion. We see minimal levels of MCH during emotion and during social interaction. However, our data show that the levels of these peptides are not always inversely related. The levels of both are minimal in pain. The major increase in MCH at sleep onset is not matched by a major decrease in Hcrt-1. Conversely, the major increase in Hcrt-1 levels at wake onset is not matched by a major decrease in MCH levels. The activity of these peptides also differed after food consumption, with a significant increase in MCH levels but no significant change in Hcrt-1 levels. A considerable amount of work has suggested that Hcrt release is linked to food intake [20] , but some recent work has raised doubts about the specificity of this relation [4] , [23] , [46] . In the current study we have directly compared the effects of eating with the effects of mood on Hcrt-1 level in humans, and found that the latter has a far greater effect on Hcrt-1 levels. Fos studies have produced conflicting conclusions regarding the determinants of Hcrt cell activation. When stress lasting for 5–30 min was followed by release back into the home cage, Fos was expressed in Hcrt neurons [47] . However, when stress was maintained for the entire 2-h incubation period for Fos expression, little or no Fos expression was observed in the Hcrt neurons [48] . Furlong et al . [49] concluded that Fos expression in Hcrt neurons was maximal during exploration, consistent with our prior data on Hcrt unit activity in the rat [11] . These data suggest that the increased Fos expression in Hcrt neurons reported in a few papers with restraint, shock or ‘panic’ [50] may be because of increased waking and grooming subsequent to the aversive stimulus, compared with controls, rather than the aversive situation itself. Furthermore, studies of CSF retrieved from the lumbar cistern [50] are difficult to interpret, as lumbar CSF levels represent an average of peptide release over the prior 6 h. Laughter, social interaction and anger are the three most frequent triggers of human cataplexy, the most debilitating symptom of narcolepsy in many patients [7] . Animal studies cannot shed much light on why this is so, as important aspects of these behaviours are qualitatively unique to humans. Our current findings show that a common element in these three behaviours in non-narcoleptic humans is a surge of Hcrt levels, a peptide that is pathologically deficient in those who have cataplexy, that is, narcoleptics [1] , [2] . Relatively little work has been done on the behavioural correlates of MCH cell activity. Studies with sleep deprivation and sleep rebound [44] suggest that MCH activity may promote sleep in accordance with the current findings. However, these cells have not yet been studied during the performance of operant tasks in waking, which might allow comparison of their discharge with Hcrt cells. In summary, we found that Hcrt-1 level, as assayed in the amygdala, was not linked to arousal per se , but was maximal during positive emotions, anger, social interaction and awakening in humans. Conditions that trigger cataplexy and high Hcrt-1 levels may be those that elicit approach. In contrast, we found that conditions associated with minimal Hcrt levels are those eliciting withdrawal, such as pain, or in the case of our prior animal work, anxiety [5] , [11] . In contrast, MCH levels were maximal during sleep onset and minimal during social interactions. Together these results suggest a previously unappreciated emotional specificity in the activation of arousal and sleep induction systems in humans. Abnormalities in the pattern of activation of these systems may contribute to a number of psychiatric disorders. Rat studies All animal studies followed the NIH guidelines and were approved by the Institutional Animal Care and Use Committee of the VA Greater Los Angeles Healthcare System. Rats were anaesthetized with a ketamine/xylazine injection (100 and 15 mg kg −1 , i.p.). Anaesthesia was maintained with 0.5–1.0% isoflurane. Using a stereotaxic frame under aseptic conditions, two guide cannulae were implanted in each rat. The cannulae tips were directly (0.5 mm) above the right hypothalamus (perifornical area; A: −3.2, L: −1.6, H: −7.5) and left amygdala (central nucleus; A: −2.5, L: 4.1, H: −7). Stainless steel screws were implanted bilaterally over the frontal and parietal areas for the EEG recording, and electromyography was recorded with stainless steel wires inserted into the dorsal neck muscles. Microdialysis probes with 2-mm membranes (Eicom probes C-I-14-02, Hospal membrane, 40 kDa cut-off) were inserted through the guide cannulae (AG-14, Eicom) into the target areas. Teflon tubing (1 mm; JT-10-100, Eicom) was connected to the inflow and outflow portions of the probe. Artificial CSF (Harvard Apparatus, MA, USA) with 0.025% rat serum albumin (Sigma) was continuously perfused at 2 μl min −1 using a syringe pump (EPS-64, Eicom). Samples were collected every 5 min using a fraction collector with an electronic cooler (EFC-82 and EFR-82, Eicom). Samples were stored at −80 °C until analysed with radioimmunoassay. Each sample was analysed for both peptides by sequential multiple-antigen solid-phase radioimmunoassay [51] , providing IC50/limit of detection of 0.6/0.025 fmol and 1.5/0.025 fmol for Hcrt-1 and MCH, respectively. To determine probe recovery, a probe similar to the ones used in this study (2 mm membrane, C-I-14-02, Eicom) was placed in solutions of 0.1, 1 and 10 n M unlabelled Hcrt-1 and MCH (Phoenix Pharmaceuticals) in artificial CSF and 0.025% rat serum albumin, and perfused at a rate of 2 μl min −1 . The in vitro recovery of Hcrt-1 and MCH across a 2.0-mm long membrane was 1.5±0.2% for Hcrt-1 ( n =4) and 3.5±0.8% for MCH ( n =4). Measured concentrations can be assumed to reflect changes in release, as well as any changes in the metabolic breakdown of the peptides. Human studies Eight patients ( Table 2 ) diagnosed with pharmacologically resistant epilepsy were studied. These patients required implantation of depth electrodes to identify the brain area generating their seizures, because presurgical diagnostic evaluation with scalp EEG, magnetic resonance imaging and positron emission tomography scans had localized no anatomically or functionally abnormal site for curative surgical resection. All patients gave their informed consent for participation in this study, and the protocol was approved by the UCLA Medical School Institutional Review Board. As the area in the brain generating seizure activity is usually quite limited, in our experience, identification and subsequent removal of the seizure focus renders the great majority of patients free from seizures for the remainder of their lives [52] . After the surgical implant, the subjects recovered in the neurological intensive care unit for approximately 24 h, and they were then transferred to the Medical–Surgical Specialty Unit where the studies were done. The depth EEG electrode was 1.25 mm in diameter and consisted of magnetic resonance imaging compatible, flexible, polyurethane probes with six or seven 1.5-mm-wide platinum contacts with intercontact separations of 1.5–4 mm ( Fig. 5a ). It was stereotaxically inserted under general anaesthesia through temporal lobe cortex into the amygdala ( Figs 1 and 5b ). The lumen of the EEG electrode allowed insertion of the microdialysis probe. The microdialysis probe consisted of two fused silica tubes used for inflow (105 and 40 μm outer diameter and inner diameter, respectively; length 39 cm) and outflow (150 and 75 μm outer diameter and inner diameter, respectively; length 39 cm; Fig. 5a ). The tubes were inserted into a 20-mm long Cuprophan (12 kDa cut-off value, 220 μm outer diameter, 200 μm inner diameter) membrane (made by Membrana GmbH, Wuppertal, Germany), or into a Hospal membrane in the case of patient d378. Dialysis membranes extended 5 mm beyond the EEG probe (Ad-Tech Medical Instrument Corp., BF-7 Macro Depth Electrode) and connected to a fraction collector via fused silica tubing (Polymicro Technologies, 375 and 150 μm outer diameter and inner diameter, respectively; length 150 cm). A mini-pump (CMA 102) was used to perfuse sterile phosphate-buffered artificial CSF through the probes at a flow rate of 1 μl min −1 . Samples were collected continuously at 15 min intervals (30 min for patient d378) for a period of 2–4 days and stored at −80 °C. The in vitro recovery of [ 125 I] Hcrt-1 with a Cuprophan membrane constructed in the same manner as those used in this study was approximately 4.5%. The recovery of Hcrt-1 and MCH as measured by radioimmunoassay with the Cuprophan probe was 2.4±0.7% for Hcrt-1 ( n =10) and 1.4±0.3% for MCH ( n =10). The actual probes used in the patients of this study could not be tested for peptide recovery, as residual peptides could trigger an immune response when implanted into the brain. These probes were tested for glutamate and aspartate or monoamines, and average recovery was found to be 29% for aspartate, 31% for glutamate, and 23, 27, and 45% for norepinephrine, dopamine, and serotonin, respectively. Our early work establishing the feasibility of measuring peptides with microdialysis [51] demonstrated that the thin-wall thickness version of the Cuprophan membrane was the optimal membrane for the current studies. A 12-kDA cut-off value is above the molecular weight of both peptides studied here (3,561 and 2,387 for Hcrt-1 and MCH, respectively). 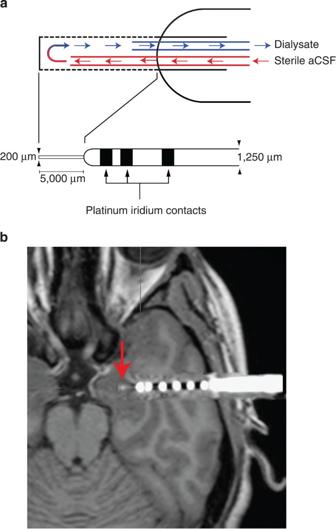Figure 5: Design and placement of electrodes. (a) Electrode contained external contacts for localizing seizure focus and internal space for a 200-μm diameter microdialysis membrane. The membrane protruded 5 mm from the outer cannula. Artificial CSF flowed in through a 105-μm outer diameter silica tube and flowed out of the Cuprophan membrane through a 150-μm outer diameter silica tube. Dialysates were collected at 15 min intervals and immediately frozen to −80°. Samples were subsequently analysed for both Hcrt-1 and MCH, using our multiple-antigen solid state radioimmunoassay51. (b) Image of implanted probe in the amygdala (metal contacts produce magnetic resonance imaging (MRI) artifact). Computed tomography image of electrode was superimposed on MRI after computer registration (alignment in three dimensions) of the two scans. Figure 5: Design and placement of electrodes. ( a ) Electrode contained external contacts for localizing seizure focus and internal space for a 200-μm diameter microdialysis membrane. The membrane protruded 5 mm from the outer cannula. Artificial CSF flowed in through a 105-μm outer diameter silica tube and flowed out of the Cuprophan membrane through a 150-μm outer diameter silica tube. Dialysates were collected at 15 min intervals and immediately frozen to −80°. Samples were subsequently analysed for both Hcrt-1 and MCH, using our multiple-antigen solid state radioimmunoassay [51] . ( b ) Image of implanted probe in the amygdala (metal contacts produce magnetic resonance imaging (MRI) artifact). Computed tomography image of electrode was superimposed on MRI after computer registration (alignment in three dimensions) of the two scans. Full size image The statistical analyses presented above included only the seven patients implanted with the Cuprophan membranes. The results with the Hospal membrane ( Fig. 4 ) were similar to those found with the Cuprophan membrane. The microdialysis procedure was also being used in these patients to sample neurotransmitter levels before and during seizures to better understand the seizure initiation process and its variation across patients [52] , [53] , [54] , [55] , [56] . We found that Hcrt and MCH levels assayed with our Cuprophan membrane were stable for as long as 4 days. We have been able to measure glutamate and glutamine with these electrodes for up to 6 days [57] . Daytime light levels averaged 1,000 lux and nighttime light levels were reduced to 50 lux. For the analysis of sleep onset, the pure wake sample preceding the transition and the following sample containing a transition to sleep were analysed. For the analysis of wake onset, the pure sleep sample preceding the transition and the following sample containing a transition to wake were analysed. State transitions were determined behaviourally. For analysis of the eating data, 60 min before and after eating were averaged to calculate peptide levels before and after eating. ‘During eating’ included all samples that contained periods of eating. Eating periods ranged from 15 to 60 min. ‘Awake’ samples were those not assigned to social interaction, emotion or sleep categories. During the period of observation, the subjects were free to walk about the room and hallways, watch television, play video games, make phone calls and receive visitors. However, most of our observations, including mood assays, eating and sleeping observations were made with the patients in bed or seated next to their bed. Our questionnaire was given to the subjects during waking at hourly intervals synchronized with the corresponding 15 min aliquot. Behaviour was scored as social interaction if the patient talked with another person or persons for at least one-third of the 15 min sample duration. Samples were scored for emotion if the patient stated a positive or negative emotion, or openly and objectively showed some emotional expression, such as laughing or crying, at least once during the sample period. Positive emotion included laughing or excitement (for example, watching a sports game and seeing the favoured team score a home run) and negative emotion included sadness or frustration. In four patients, mood was also assessed with the questionnaire ( Supplementary Methods ) presented at hourly intervals. All behavioural judgments were recorded before the analysis of the samples. The samples used in the present study were all derived from amygdala electrodes that physiological analysis determined not to be an independent seizure focus. All data were collected during periods free of seizures. Statistical analysis Data with multiple comparisons were analysed with one-way analysis of variance and Fisher’s least significant difference post-hoc comparisons after normalization and log transformation (GB-Stat, Silver spring, MD, USA). Table 3 presents the number of samples for each category along with means and standard error of the mean. Correlation studies of anger and pain were calculated across trials. Statistical significance of all findings was determined by P <0.05. How to cite this article: Blouin, A.M. et al . Human hypocretin and melanin-concentrating hormone levels are linked to emotion and social interaction. Nat. Commun. 4:1547 doi: 10.1038/ncomms2461 (2013)